Optical freezing of charge motion in an organic conductor Dynamical localization, that is, reduction of the intersite electronic transfer integral t by an alternating electric field, E ( ω ), is a promising strategy for controlling strongly correlated systems with a competing energy balance between t and the Coulomb repulsion energy. Here we describe a charge localization induced by the 9.3 MV cm −1 instantaneous electric field of a 1.5 cycle (7 fs) infrared pulse in an organic conductor α-(bis[ethylenedithio]-tetrathiafulvalene) 2 I 3 . A large reflectivity change of >25% and a coherent charge oscillation along the time axis reflect the opening of the charge ordering gap in the metallic phase. This optical freezing of charges, which is the reverse of the photoinduced melting of electronic orders, is attributed to the ~10% reduction of t driven by the strong, high-frequency ( ω ≧ t / ħ ) electric field. Ultrafast control of conduction and magnetic properties in strongly correlated systems [1] , [2] , [3] has been extensively studied from the perspective of photoinduced insulator-to-metal transitions, or, equivalently, the ‘melting’ of electronic orders (red arrow in Fig. 1a ) in Mott insulators [4] , [5] , [6] , [7] , [8] , [9] , [10] , charge-ordered (CO) systems [11] , [12] , [13] , [14] and charge/spin density wave materials [6] , [15] , [16] , [17] , [18] , [19] , [20] . Recently, the excitation of coherent phonons has been established as a leading strategy for the melting/constructing of electronic orders [8] , [9] , [15] , [16] , [17] , [18] , [19] , [20] . On the other hand, the development of strong electric fields (>MV cm −1 ) of few-cycle optical pulses and recent theoretical studies using dynamical mean-field theory suggest that extreme non-equilibrium electronic states, such as Floquet states, negative temperatures and superconducting states [21] , [22] , can be achieved. 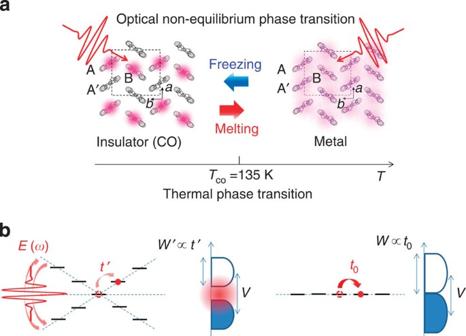Figure 1: Melting and freezing of charge motion in α-(ET)2I3and AC-field-induced charge localization. (a) CO insulator-to-metal transition (red arrow, melting) and metal-to-CO insulator transition (blue arrow, freezing) for both thermal (equilibrium) and optical (non-equilibrium) transitions in α-(ET)2I3. (b) CO gap is opened by the decrease of transfer integralt, because of the competing energy balance between Coulomb interactionVandt.tis changed fromt0tot', induced by the strong AC electric fieldE(ω). Figure 1: Melting and freezing of charge motion in α-(ET) 2 I 3 and AC-field-induced charge localization. ( a ) CO insulator-to-metal transition (red arrow, melting) and metal-to-CO insulator transition (blue arrow, freezing) for both thermal (equilibrium) and optical (non-equilibrium) transitions in α-(ET) 2 I 3 . ( b ) CO gap is opened by the decrease of transfer integral t , because of the competing energy balance between Coulomb interaction V and t . t is changed from t 0 to t' , induced by the strong AC electric field E ( ω ). Full size image In highly non-equilibrium phenomena, reducing the intersite transfer integral t by modulating the site energy under strong continuous-wave (CW) [21] , [23] , [24] , [25] , [26] and pulsed [22] , [26] alternating current (AC) fields E ( ω ), shown in Fig. 1b , plays an important role. Such an intense modulation of the electronic structure driven by a strong electric field, referred to as ‘dynamical localization’, provides a new strategy for controlling charge motion in strongly correlated materials, which have a competing energy balance between the on-site or intersite Coulomb repulsion and t (ref. 27 ). Our target material is a layered organic conductor, α-(ET) 2 I 3 (ET: bis[ethylenedithio]-tetrathiafulvalene), which exhibits a thermal (equilibrium) metal-to-CO insulator transition at T CO =135 K (refs 28 , 29 , 30 , 31 , 32 ) and a photoinduced (non-equilibrium) transition [14] as illustrated in Fig. 1a . Efficient photoinduced insulator-to-metal transitions of >200 ET molecules/photon have previously been demonstrated [14] . However, the optical response of the metallic phase at T > T CO remains unclear. In this study, we perform pump-probe transient reflectivity measurements for the metallic phase of α-(ET) 2 I 3 using 7 fs 1.5 cycle infrared pulses. Our results demonstrate the optical freezing of charges or, equivalently, photoinduced charge localization in the metallic phase (blue arrow in Fig. 1a ). We discuss the mechanism on the basis of theories that have been proposed for non-equilibrium states generated by high-frequency CW and pulsed AC fields. Thermal metal-to-CO insulator transitions The optical conductivity in the mid- and near-infrared region in Fig. 2a has a clear opening of the CO gap at ~0.1–0.2 eV and a spectral weight transfer to a higher energy at the thermal metal-to-insulator transition [29] , [30] . 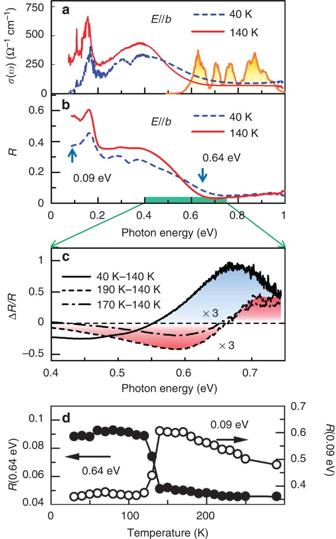Figure 2: Steady-state optical conductivity and reflectivity spectra. (a) Optical conductivity (σ) spectra of α-(ET)2I3at 40 K (CO: dashed blue curve) and at 140 K (metal: solid red curve). The spectrum of the 7 fs pulse is indicated by the orange curve. (b) Reflectivity (R) spectra at 40 K (CO) and at 140 K (metal). (c) The spectra for three temperature differentials: [R(40 K)−R(140 K)]/R(140 K) (solid curve with blue shading), [R(190 K)−R(140 K)]/R(140 K) (dashed curve ( × 3) with red shading) and [R(170 K)−R(140 K)]/R(140 K) (dashed–dotted curve ( × 3)). (d) Reflectivities measured at 0.09 and 0.64 eV (indicated by the blue arrows on the spectrum inb), plotted as a function of temperature. Figure 2b shows the steady-state reflectivity ( R ) at 140 K (metal: solid red curve) and 40 K (CO: dashed blue curve). As shown in Fig. 2d , at T CO , R abruptly decreases for 0.09 eV (open circles) and increases for 0.64 eV (closed circles) as the temperature decreases. Such a large change (80% at 0.64 eV, 60% at 0.09 eV) in R at the metal-to-insulator transition directly corresponds to the opening of the CO gap and the transfer of the spectral weight to a higher energy of the optical conductivity [29] , [30] , as shown in Fig. 2a . Figure 2c shows the spectral differences at different temperatures. The solid curve shows [ R (40 K)− R (140 K)]/ R (140 K), reflecting the metal-to-insulator change across T CO . The dashed and dashed–dotted curves show [ R (190 K)− R (140 K)]/ R (140 K) and [ R (170 K)− R (140 K)]/ R (140 K), exhibiting increases in the electron-lattice temperature up to 190 and 170 K, respectively. Thus, the marked increase of R at >0.55 eV (blue shading) clearly characterizes the metal-to-insulator change across T CO , whereas the rise of the electron-lattice temperature is detected as a reflectivity decrease below 0.65 eV. Figure 2: Steady-state optical conductivity and reflectivity spectra. ( a ) Optical conductivity ( σ ) spectra of α-(ET) 2 I 3 at 40 K (CO: dashed blue curve) and at 140 K (metal: solid red curve). The spectrum of the 7 fs pulse is indicated by the orange curve. ( b ) Reflectivity ( R ) spectra at 40 K (CO) and at 140 K (metal). ( c ) The spectra for three temperature differentials: [ R (40 K)− R (140 K)]/ R (140 K) (solid curve with blue shading), [ R (190 K)− R (140 K)]/ R (140 K) (dashed curve ( × 3) with red shading) and [ R (170 K)− R (140 K)]/ R (140 K) (dashed–dotted curve ( × 3)). ( d ) Reflectivities measured at 0.09 and 0.64 eV (indicated by the blue arrows on the spectrum in b ), plotted as a function of temperature. 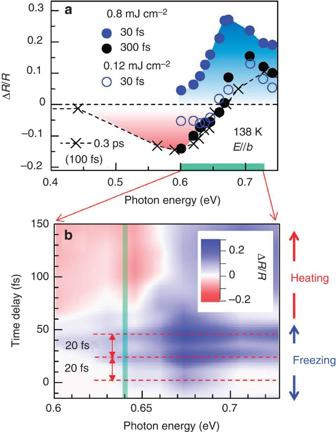Figure 3: Transient reflectivity spectra and their time evolutions. (a) Transient reflectivity (ΔR/R) spectra forIex=0.8 and 0.12 mJ cm−2attd=30 fs (closed blue circles forIex=0.8 mJ cm−2, open blue circles forIex=0.12 mJ cm−2) and 300 fs (closed black circles forIex=0.8 mJ cm−2) after excitation by a 7-fs pulse. ΔR/Rattd=300 fs after a 100-fs pulse excitation forIex=0.8 mJ cm−2is shown as the crosses. (b) Temporal change of the ΔR/Rspectrum, plotted as a two-dimensional (probe energy–delay time) map. Positive and negative ΔR/Rare shown by the blue and red shadings, respectively. Full size image Photoinduced charge localization Figure 3a shows the transient reflectivity (Δ R / R ) spectra for time delays ( t d ) of 30 fs (closed blue circles for an excitation intensity I ex =0.8 mJ cm −2 , open blue circles for I ex =0.12 mJ cm −2 ) and 300 fs (closed black circles for I ex =0.8 mJ cm −2 ) after excitation by a 7-fs pulse covering the spectral range 0.6–0.95 eV. The spectrum shown by crosses represents Δ R / R at t d =300 fs after a 100-fs pulse excitation for I ex =0.8 mJ cm −2 . A large increase of R (Δ R / R =0.28 at 0.66 eV) was observed at t d =30 fs for I ex =0.8 mJ cm −2 , as shown by the blue shading in Fig. 3a . The spectral shape of Δ R / R is analogous to that of the temperature differential spectrum [ R (40 K)− R (140 K)]/ R (140 K) in Fig. 2c , suggesting that a photoinduced metal-to-insulator change occurred. In contrast, as shown by the crosses, the black closed circles and the red shading, the spectral shapes and the magnitude of Δ R / R measured at t d =300 fs are analogous to the differential spectrum [ R (190 K)− R (140 K)]/ R (140 K), reflecting an increase in the electron-lattice temperatures up to 190 K. In such a time domain (300 fs), the lattice system cannot be thermalized and a quasi-thermalized state is formed as a result of the interaction between the charge and various short-period vibrational and optical phonon modes. Therefore, the lattice temperature shown in the reflectivity spectrum at t d =300 fs can be defined as a local temperature consisting solely of short-period modes. For I ex =0.12 mJ cm −2 , the Δ R / R spectrum shown by the open blue circles indicates that the metal-to-charge-localized change does not occur under weak excitation conditions. Figure 3: Transient reflectivity spectra and their time evolutions. ( a ) Transient reflectivity (Δ R / R ) spectra for I ex =0.8 and 0.12 mJ cm −2 at t d =30 fs (closed blue circles for I ex =0.8 mJ cm −2 , open blue circles for I ex =0.12 mJ cm −2 ) and 300 fs (closed black circles for I ex =0.8 mJ cm −2 ) after excitation by a 7-fs pulse. Δ R / R at t d =300 fs after a 100-fs pulse excitation for I ex =0.8 mJ cm −2 is shown as the crosses. ( b ) Temporal change of the Δ R / R spectrum, plotted as a two-dimensional (probe energy–delay time) map. Positive and negative Δ R / R are shown by the blue and red shadings, respectively. Full size image Charge-ordering gap oscillation along the time axis The temporal change of the Δ R / R spectrum is plotted as a two-dimensional (probe energy—delay time) map in Fig. 3b . Positive and negative Δ R / R are shown by the blue and red shadings, respectively. The spectrum for t d <50 fs, reflecting the transient CO state, oscillates with a period of 20 fs as indicated by the red dotted lines. Then, the spectral shape of Δ R / R markedly changes with the melting of the transient CO and the increase of electron/lattice temperatures shown as the red area in the time scale of 50–100 fs. Such spectral change occurs simultaneously as the oscillation decays. The time profile of Δ R / R sliced at 0.64 eV is shown in Fig. 4a . A positive Δ R / R (solid curve with blue shading) at I ex =0.8 mJ cm −2 persists for t d =50 fs after the excitation pulse. Then, Δ R / R becomes negative (red shading), indicating that the photoinduced CO state collapsed because of the increase of electron-lattice temperature. In contrast, for I ex =0.12 mJ cm −2 , a positive signal was not detected at 0.64 eV, as shown by the dashed–dotted curve. It is worth noting that the time profile was modulated by the oscillating component with a period of 20 fs. This oscillation, shown in Fig. 4b , can be attributed to the intermolecular charge oscillation reflecting the CO gap, because the time-resolved spectrum of the oscillating component at t d =0–40 fs obtained by the wavelet (WL) analysis (blue curve, inset of Fig. 4b ) corresponds to the optical conductivity spectrum near the CO gap of ~0.1 eV at 10 K (black curve in the inset). 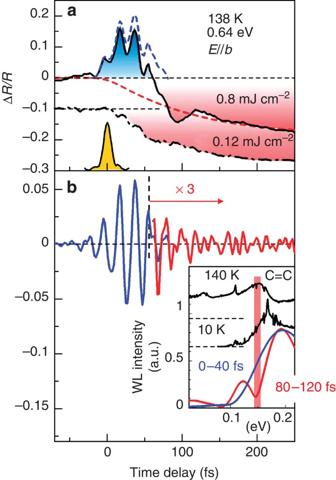Figure 4: Time profiles of transient reflectivity measured at 0.64 eV. (a) Time evolution of transient reflectivity (ΔR/R) observed at 0.64 eV forIex=0.8 mJ cm−2(solid curve) and 0.12 mJ cm−2(dashed–dotted curve). The cross-correlation between the pump and the probe pulses is also indicated by the orange shading. The dashed blue curve shows the positive component of ΔR/R, reflecting the photoinduced charge localization, which was estimated assuming that the negative component grows exponentially (dashed red curve). (b) Oscillating component of the time profile. The time-resolved spectra of the oscillating component obtained by wavelet (WL) analysis (blue curve for 0–40 fs, red curve for 80–120 fs) are shown in the inset. Optical conductivity spectra at 10 K (CO) and 140 K (metal) are shown by the black curves in the inset. Figure 4: Time profiles of transient reflectivity measured at 0.64 eV. ( a ) Time evolution of transient reflectivity (Δ R / R ) observed at 0.64 eV for I ex =0.8 mJ cm −2 (solid curve) and 0.12 mJ cm −2 (dashed–dotted curve). The cross-correlation between the pump and the probe pulses is also indicated by the orange shading. The dashed blue curve shows the positive component of Δ R / R , reflecting the photoinduced charge localization, which was estimated assuming that the negative component grows exponentially (dashed red curve). ( b ) Oscillating component of the time profile. The time-resolved spectra of the oscillating component obtained by wavelet (WL) analysis (blue curve for 0–40 fs, red curve for 80–120 fs) are shown in the inset. Optical conductivity spectra at 10 K (CO) and 140 K (metal) are shown by the black curves in the inset. Full size image Although the C=C vibration energy is near the CO gap [29] , [30] , the vibrational contribution can be detected separately after t d >50 fs, that is, the wavelet spectra at t d =80–120 fs indicated by the red curve in the inset of Fig. 4b shows a dip at ~0.15 eV (which equals the vibration peak of the optical conductivity at 140 K (refs 29 , 30 ) in the inset) reflecting the destructive interference between charge motion and vibration [33] . Therefore, the intense 20 fs oscillation detected before the appearance of the charge-vibration interference dip is attributed to the oscillation of the CO gap. Such CO gap oscillation has been detected in the precursor step to the CO melting [33] , although the amplitude was much smaller (<1% of the Δ R / R signal) than the present case. Because of the ultrafast decay within 50 fs (corresponding to the energy scale of ħ /50 fs=0.08 eV) of the photoinduced state, we cannot verify the insulating gap below 0.1 eV. However, the gap-like spectral shape at 0.1–0.2 eV, as described above, clearly indicates that the charge motion on the corresponding energy scale is frozen as if the charge distribution on the ET molecules were analogous to that in the CO insulator. In this limited sense, the CO gap is regarded as opened. Considering that the charge-vibration interference dip appears after the photoinduced charge localization occurs, the vibration-induced mechanism is ruled out, that is, the charge localization is driven by the electronic interaction, although vibration may play some role in stabilizing the transient CO state. Here the lifetime of the transient CO state (<50 fs) is much shorter than that of the coherent phonon-induced state (~1 ps or longer), which has been reported as the melting of a Mott insulator [8] , [9] or the ordering of the transient spin density wave [19] , [20] . Such a short lifetime indicates that the transient CO state is not adequately stabilized by vibrational and lattice motions. From Δ R / R =0.28 at 0.64 eV and the temperature difference [ R (40 K)− R (140 K)]/ R (140 K)=0.8 at the same energy, the volume fraction of the photoinduced CO state is evaluated to be ~35%. As I ex =0.8 mJ cm −2 corresponds to ~0.0145 photons/ET molecule, the efficiency of this process is 25 ET/photon. This is much lower than that for photoinduced melting of the CO state(>200 ET/photon [14] ), demonstrating that the mechanism of the photoinduced charge localization is completely different from that of the insulator-to-metal transition. 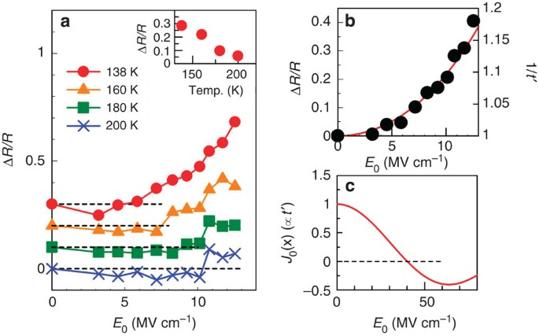Figure 5: Electric field and temperature dependences of transient reflectivity. (a) Transient reflectivity (ΔR/R) at 0.64 eV as a function of electric fieldfor various temperatures. Inset: temperature dependence of ΔR/RatE0=11.7 MV cm−1. (b) Positive component of ΔR/Rderived by subtracting the negative component (see text) as a function ofE0, together with 1/t'in units oft0(E0<13 MV cm−1) calculated from equation 1 (solid red curve). (c) Zeroth-order Bessel functionJ0∝t' as a function ofE0. Figure 5a shows Δ R / R at 0.64 eV as a function of the instantaneous electric field for various temperatures. An increase in R (positive Δ R / R ) is detectable only for I ex >0.31 mJ cm −2 ( E 0 =5.8 MV cm −1 ) at 138 K, whereas the negative Δ R / R for I ex <0.31 mJ cm −2 is due to the rise in the electron-lattice temperature. As shown in the inset, the efficiency of the photoinduced charge localization becomes larger near T CO . We can evaluate the positive component of Δ R / R by subtracting the negative component of the time profile shown in Fig. 4a , assuming that the negative component grows exponentially along the time axis (the dashed red curve in Fig. 4a ). The resultant positive component exhibits a nonlinear increase as a function of E 0 , as shown in Fig. 5b . Figure 5: Electric field and temperature dependences of transient reflectivity. ( a ) Transient reflectivity (Δ R / R ) at 0.64 eV as a function of electric field for various temperatures. Inset: temperature dependence of Δ R / R at E 0 =11.7 MV cm −1 . ( b ) Positive component of Δ R / R derived by subtracting the negative component (see text) as a function of E 0 , together with 1/ t' in units of t 0 ( E 0 <13 MV cm −1 ) calculated from equation 1 (solid red curve). ( c ) Zeroth-order Bessel function J 0 ∝ t ' as a function of E 0 . Full size image In non-equilibrium states induced by a strong AC field E ( ω ), t is reduced for CW [21] , [23] , [24] , [25] and pulsed [22] , [26] light. According to the dynamical localization theory [23] , [24] , [25] , [26] for a CW AC field, the effective t (= t ′) can be represented as, where t 0 is the transfer integral for zero field. Here, Ω AB ≡ e r AB · E 0 / ħ , where E 0 and ω , respectively, denote the amplitude and angular frequency of the electric field of the light; E ( t )= E 0 sin( ωt ); r AB is the vector from the A site to its nearest-neighbour B site of α-(ET) 2 I 3 , as shown in Fig. 1a ; and e is the elementary charge. Equation (1) is satisfied for CW light. In addition, on the basis of the numerical solution of the time-dependent Schrödinger equation for the two-site tight-binding model and a model for a CO molecular conductor [26] , this relation has recently been shown to be satisfied by pulsed light, with respect to the efficiency of the intersite electronic transition (that is, the energy increment due to the pulsed light). Also, in the dynamical mean-field theory calculations, the change in the electronic state into one with modified t appears within the time scale of a few optical cycles after the sudden application of a CW AC field [21] . This fact also suggests that the dynamical localization functions transiently with the few-cycle pulse. If we use the parameter r AB cos θ =5.4 angstroms (refs 34 , 35 ); where θ represents the relative angle between r AB and E , t is reduced, as it is proportional to the zeroth order Bessel function J 0 , and becomes zero at 40 MV cm −1 (Ω AB / ω =2.40), as shown in Fig. 5c . From Fig. 5c , we can estimate that the change in J 0 ∝ t ′ is approximately 10% for a typical instantaneous field of 9.3 MV cm −1 ( I ex =0.8 mJ cm −2 ). To demonstrate the instability of the metallic phase induced by this 10% change in t , we roughly estimated the change of T CO by changing t . 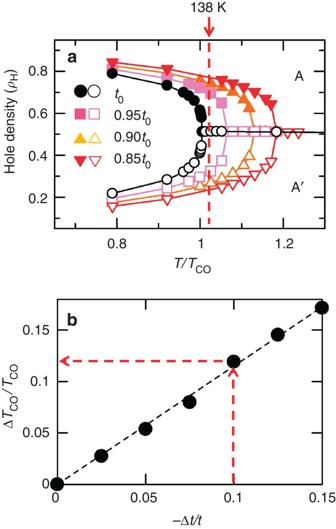Figure 6: Changes of transition temperature by reducing transfer integral. (a) The hole densities (ρH) at the A and A' molecules inFig. 1aas a function of the normalized temperatureT/TCO, calculated using the Hartree–Fock approximation for an extended Hubbard model36fort0, 0.95t0, 0.9t0and 0.85t0(circles, squares, triangles and inverted triangles, respectively). (b) Change inTCO(=ΔTCO/TCO) as a function of decreasing transfer integralt(−Δt/t) shown by the black closed circles. The dashed line serves as a guide to the eye. The dashed red arrows indicate that a 10% reduction intcauses a 12% increase inTCO. Figure 6a shows the temperature dependence of the hole densities ( ρ H ) at the A and A′ molecules in Fig. 1a as a function of the normalized temperature T / T CO , calculated using the Hartree–Fock approximation for an extended Hubbard model [36] . A charge disproportionation occurs below T / T CO =1, as indicated by the closed (A: charge rich) and open (A′: charge poor) circles for the original t 0 . We also calculated the ρ H versus T / T CO relation with changing t , where the rectangles, upward triangles and downward triangles show the calculated values for 0.95 t 0 , 0.9 t 0 and 0.85 t 0 , respectively. Figure 6b illustrates that the change in T CO (=Δ T CO /T CO ) is proportional to the decrease in t (=−Δ t / t ), indicating that a 10% change in t causes a 12% change in T CO from 135 to 152 K. Thus, T CO increases across the measured temperature (138 K). Figure 6: Changes of transition temperature by reducing transfer integral. ( a ) The hole densities ( ρ H ) at the A and A' molecules in Fig. 1a as a function of the normalized temperature T / T CO , calculated using the Hartree–Fock approximation for an extended Hubbard model [36] for t 0 , 0.95 t 0 , 0.9 t 0 and 0.85 t 0 (circles, squares, triangles and inverted triangles, respectively). ( b ) Change in T CO (=Δ T CO /T CO ) as a function of decreasing transfer integral t (−Δ t / t ) shown by the black closed circles. The dashed line serves as a guide to the eye. The dashed red arrows indicate that a 10% reduction in t causes a 12% increase in T CO . Full size image For our experimental conditions (<12 MV cm −1 ), 1/ t′ (in units of 1/ t 0 ) shows a nonlinear dependence on E 0 (red curve in Fig. 5b ). This nonlinear dependence of 1/ t ′ on E 0 is consistent with the relation between Δ R / R and E 0 (closed circles in Fig. 5b ). Considering that R reflects the metal-to-insulator transition ( Fig. 2b ), it is reasonable to assume that Δ R / R is proportional to the efficiency of the transient charge localization. As such, the E 0 dependence of Δ R / R , can be described by 1/ t′ . According to recent studies on sub-cycle asymmetric pulses [22] , the momentum shift of the band structure is given by the ‘dynamical phase’ φ =∫ dtE ( t ) (ref. 22 ). However, in the present case, this is estimated to be φ =1.66 × 10 −4 [rad] at most, which is much smaller than φ = π /2[rad], and is too small to cause a detectable momentum shift. Such shift would be detected if the width of the asymmetric pulse were shorter than ~3 fs at this wavelength. Another problem lies in the mechanism driving the reduced t , which should be applicable to events before the excitation ends, that is, ~7 fs. The reason why the photoinduced CO persists for ~50 fs after the 7 fs pulse is unclear at the moment. Further experiments and theoretical considerations will be needed to clarify this issue. In summary, this report demonstrates a large reflectivity increase (>25%) and a coherent CO gap oscillation along the time axis indicating the opening of a CO gap by the 9.3 MV cm −1 electric field of a 1.5 cycle, 7 fs near-infrared pulse in an organic conductor α-(ET) 2 I 3 . The plausible mechanism for such a dramatic change in the electronic state is the reduction of t (~10%) driven by this strong high-frequency field. Sample preparation Single crystals of α-(ET) 2 I 3 (2 × 1 × 0.1 mm) were prepared using a method described in a previous study [28] . 7-fs Infrared pulse generation A broadband infrared spectrum for the 7-fs pulse covering 1.2–2.3 μm, shown by the orange curve in Fig. 2a , was obtained by focusing a carrier-envelope phase stabilized idler pulse (1.7 μm) from an optical parametric amplifier (Quantronix HE-TOPAS pumped by Spectra-Physics Spitfire-Ace) onto a hollow fibre set within a Kr-filled chamber (Femtolasers). Pulse compression was performed using both active mirror (OKO Technologies, 19-ch linear MMDM) and chirped mirror (Femtolasers, Sigma-Koki) techniques. The pulse width derived from the autocorrelation of the generated second harmonic was 7 fs, which corresponds to 1.5 optical cycles. The instantaneous electric field on the sample surface (excitation diameter 200 μm) for a typical excitation intensity can be evaluated as , where I peak =1.14 × 10 11 W cm −2 represents the peak power for an excitation intensity I ex of 0.8 mJ cm −2 . Transient reflectivity measurements We performed transient reflectivity experiments using both 7 and 100 fs pulses. The excitation photon energies for 7 and 100 fs pulses were 0.6–0.95 eV (7 fs) and 0.89 eV (100 fs), respectively. In the transient reflectivity measurement using a 7-fs pulse, the probe pulse reflected from the sample was detected by InGaAs detector (New-Focus model 2034) after passing through a spectrometer (Bunkoukeiki, M10). The pump-on and pump-off were alternately switched by the feed-back-controlled optical chopper (New Focus, Model 3501), synchronized with the laser driver. Each probe shot was sampled using boxcar integrators (Stanford Research, SR250). After normalization by a reference pulse, the observed intensity of respective shots was recorded in the PC. How to cite this article : Ishikawa, T. et al. Optical freezing of charge motion in an organic conductor. Nat. Commun. 5:5528 doi: 10.1038/ncomms6528 (2014).